Three-dimensional plasmonic stereoscopic prints in full colour Metal nanostructures can be designed to scatter different colours depending on the polarization of the incident light. Such spectral control is attractive for applications such as high-density optical storage, but challenges remain in creating microprints with a single-layer architecture that simultaneously enables full-spectral and polarization control of the scattered light. Here we demonstrate independently tunable biaxial colour pixels composed of isolated nanoellipses or nanosquare dimers that can exhibit a full range of colours in reflection mode with linear polarization dependence. Effective polarization-sensitive full-colour prints are realized. With this, we encoded two colour images within the same area and further use this to achieve depth perception by realizing three-dimensional stereoscopic colour microprint. Coupled with the low cost and durability of aluminium as the functional material in our pixel design, such polarization-sensitive encoding can realize a wide spectrum of applications in colour displays, data storage and anti-counterfeiting technologies. Optical resonances of metallic nanostructures have shown extraordinary capabilities in manipulating visible light in subdiffraction-limited volumes [1] , [2] , [3] , [4] , [5] , [6] . This feature enables high-density information encoding using nanostructures that resonate at different wavelengths, as seen in colour prints with resolutions at the diffraction limit of light [7] , [8] . By extending this spectral tunability to asymmetric nanostructures, resonances can be tailored to depend on the polarization of incident illumination, for example, linear [9] , [10] , [11] , [12] , [13] and circular polarizations [14] . Indeed, nano-arrays consisting of gratings [9] , [10] and cross-shaped antennas [11] have been designed to generate colour variations under orthogonal polarizations of incident light. Such polarization-dependent spectral control is highly attractive for high-density optical data storage, as demonstrated in single and multiple data layers that individually resonate at a particular wavelength or polarization of light [15] , [16] , [17] . Towards the goal of increasing information density coupled with an easy read-out, it is highly advantageous to devise independently tunable elements at the optical diffraction limit [8] , with distinct colour changes under orthogonally polarized light. Challenges, however, remain in producing microprints using a compact, single-layer architecture that can simultaneously achieve full-spectral control and polarization dependence of the scattered light. For instance, grating structures are insufficient as they support colour generation only for a single polarization [9] , [10] , for example, when the electric field is polarized perpendicular to the axis of the slit/groove. To achieve a broad spectrum of polarization-dependent colours, it is crucial to consider geometries that can fully utilize both orthogonal polarizations for colour generation, that is, individual geometries that can generate distinct colours under each polarization. In this work, we demonstrate the utility of polarization-sensitive colour prints that can encode two sets of information within the same area and further use this to produce three-dimensional (3D) stereoscopic colour microprints. We produce a stereoscopic image using reflective plasmonic colour prints, which differs from conventional passive prints for which 3D glasses comprising filters of red and green must be used. In addition to high-density multiplexed optical data storage, such polarization-dependent multicolour nanostructures could lead to ultra-high-resolution 3D displays, holograms [14] , [18] , [19] , [20] , [21] and advanced elements for anti-counterfeiting and steganography [22] . Overview of experimental setup Here, we present a single-data-layer architecture of aluminium nanostructures where each individual structure can exhibit a full range of colours in reflection mode with linear polarization dependence as depicted in the schematic of Fig. 1 . As a proof-of-concept, we demonstrate that these pixels allow for two distinct images to be embedded within a single, full-colour print, where each image can only be revealed under the intended polarized illumination. To highlight the potential of this design for high-resolution 3D full-colour elements, we further demonstrate a stereoscopic plasmonic colour microprint. A stereoscopic image was achieved from a flat sample by overlaying two laterally displaced views of an image onto the same area. Viewing the microprint through polarizers placed in the path of the microscope eyepieces revealed a different image for each polarization as the microprint is decoupled through the polarizers as illustrated in the schematic of Fig. 1d . The two separate optical paths of the microprint are thus observed and interpreted by the viewer as a 3D object. 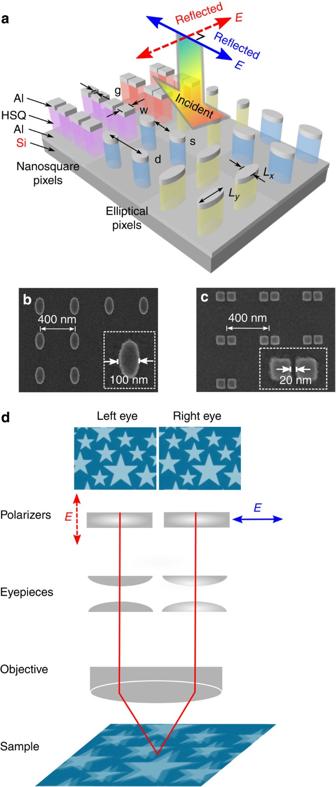Figure 1: Schematics for polarization-dependent plasmonic colour printing and stereomicroscopy. (a) White light interaction with elliptical and coupled nanosquare pixels where distinct wavelengths of light are scattered back in orthogonal polarizations as different colours from nanostructures within each individual pixel. Colour and polarization information are encoded in theLxandLydimensions (ellipses), and widthswand gap sizesg(nanosquares) spacedsapart (centre-to-centre periodd). (b,c) SEM images of (b) ellipses and (c) nanosquares. Insets: enlarged images of single pixels. (d) Schematic of a stereomicroscope setup. By adding polarizers to the eyepieces of a bright-field microscope, the imaging of two superposed microprints encoded in orthogonally polarized pixels present two laterally displaced images to the left and right eyes of a viewer, resulting in depth perception. Figure 1: Schematics for polarization-dependent plasmonic colour printing and stereomicroscopy. ( a ) White light interaction with elliptical and coupled nanosquare pixels where distinct wavelengths of light are scattered back in orthogonal polarizations as different colours from nanostructures within each individual pixel. Colour and polarization information are encoded in the L x and L y dimensions (ellipses), and widths w and gap sizes g (nanosquares) spaced s apart (centre-to-centre period d ). ( b , c ) SEM images of ( b ) ellipses and ( c ) nanosquares. Insets: enlarged images of single pixels. ( d ) Schematic of a stereomicroscope setup. By adding polarizers to the eyepieces of a bright-field microscope, the imaging of two superposed microprints encoded in orthogonally polarized pixels present two laterally displaced images to the left and right eyes of a viewer, resulting in depth perception. Full size image In our previous work, we demonstrated colour printing at the optical diffraction limit with isolated gold/silver nanodisks [8] , forming pixels that were insensitive to polarization or viewing angles [10] , [23] . In order to enhance the shelf-life and durability of pixels, aluminium was specifically chosen in our pixel design. While not as favoured as gold or silver, owing to its appreciable losses in the infrared regime (>800 nm; refs 24 , 25 ), the uniform reflectivity of aluminium in the visible spectrum makes it particularly suitable for colour-printing applications [26] , [27] . Furthermore, its inherent formation of a thin (~2–3 nm) oxide layer that causes redshifts in the spectra [28] , and a reduction of sensitivity in applications such as Raman spectroscopy, is beneficial in colour printing. The self-limiting oxide acts to significantly increase the shelf-life of the colour prints without additional barrier layers beyond the couple of weeks seen in silver [27] . Arrays of nanoposts with a height of ~95 nm were patterned in hydrogen silsesquioxane (HSQ), a negative-tone resist, by electron beam lithography (EBL) as detailed in the Methods section. Thereafter, a 20-nm aluminium layer was deposited using electron beam evaporation. It should be noted that variations in the thickness of the aluminium layer between 15 to 30 nm did not generate any visible colour changes. As the nanoposts were ~5 times taller than the thickness of the deposited metal, the metals atop the nanoposts formed isolated antennas with distinct plasmon resonances. These resonances affect the scattering of specific wavelengths in the visible spectrum and exhibit reflective colours when observed under an optical microscope. The characteristic resonance and associated colour can be controlled by tuning the shape and physical dimensions of each nanostructure [8] . Polarization-sensitive colour generation from biaxial pixels We identified the decoupling of colour and polarization as one of the challenges to achieve minimal ‘cross-talk’ between information encoded within two orthogonal polarizations. Cross-talk refers to the incomplete suppression of colours intended for one polarization when observed in the orthogonal polarization, and results in the undesired mixing of colours over an image. To realize distinct colours under orthogonally polarized illuminations and to minimize pixel cross-talk, we investigated the cross-talk and the colour range of ‘biaxial’ pixels composed of ellipses ( Fig. 1b ) and coupled nanosquare dimers ( Fig. 1c ) that can be independently varied in size, shape and orientation. By minimizing the cross-talk while generating a broad colour spectrum, one would be able to encode two sets of information within a single layer on a substrate. In contrast to nanodisks that are polarization independent [8] , an elliptical nanostructure pixel with dissimilar major and minor axes of L x and L y exhibits plasmonic resonances at different wavelengths for each axis. This biaxial symmetry generates different colours, where each pixel scatters distinct colours in orthogonal polarizations. As expected, as the ellipse evolves into a disk, its spectral response and colour becomes identical in both axes with no polarization dependence [8] . Bright-field optical images and reflection spectra measurements were obtained to investigate the optical responses of the fabricated pixels. Ellipse dimensions were systematically varied from 100 to 190 nm along both axes in 10 nm increments to investigate the full palette of colours that can be achieved. Optical micrographs of the colours generated from these dimensions for incident light polarized along the x and y axes are shown in Fig. 2a,b . Colour variations were verified by experimental ( Fig. 2c,d ) reflection spectra for the top-most row ( L y =190 nm) of the colour palette (highlighted by the dotted lines in Fig. 2a,b ). Additional spectra are shown in Supplementary Fig. 1 . 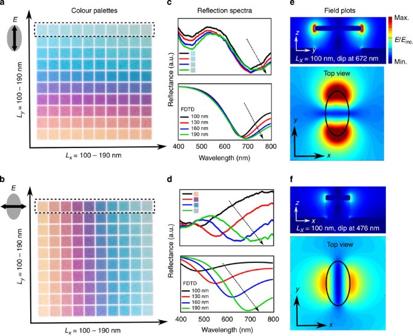Figure 2: Optical micrographs and spectral analyses for elliptical pixels with varying dimensionsLxandLy. (a,b) Optical images of colour palettes illuminated undery- andx-polarized light. Each 8 × 8 μm pixel array was spaced 1 μm away from the neighbouring pixel and comprised a square lattice of 20 × 20 nanoposts with periodd=400 nm. (c,d) Measured and simulated reflection spectra under orthogonal illumination where arrows indicate increasingLx. (e,f) Electric field enhancement plots (Ly=190 nm,Lx=100 nm). Panelsa,c,eandb,d,fcorrespond to results obtained undery- andxpolarization, respectively. Figure 2: Optical micrographs and spectral analyses for elliptical pixels with varying dimensions L x and L y . ( a , b ) Optical images of colour palettes illuminated under y - and x -polarized light. Each 8 × 8 μm pixel array was spaced 1 μm away from the neighbouring pixel and comprised a square lattice of 20 × 20 nanoposts with period d =400 nm. ( c , d ) Measured and simulated reflection spectra under orthogonal illumination where arrows indicate increasing L x . ( e , f ) Electric field enhancement plots ( L y =190 nm, L x =100 nm). Panels a , c , e and b , d , f correspond to results obtained under y - and x polarization, respectively. Full size image In the colour swatches along the diagonal of the palettes ( Fig. 2a,b ), pixels comprise symmetric nanostructures with identical L x and L y , that is, nanodisks with diameters varying from 100 to 190 nm in 10 nm increments. Therefore, no polarization-induced colour change is expected. For the off-diagonal colour swatches, distinct colours were generated when the pixels were illuminated under orthogonally polarized light. For example, a pixel comprising ellipses with L x =130 nm and L y =190 nm appeared green under y -polarized illumination and purple under x -polarized illumination. In general, when light is polarized along the dimension that was varied, that is, vertical columns under y -polarized illumination and horizontal rows under x -polarized illumination, distinct colour changes are observed for increasing dimensions. Simulated reflection spectra also show comparable trends with corresponding experimental spectra, where the spectral dips (resonances) are redshifted for each 10 nm increment, allowing the resonances to be tuned across the entire visible spectrum ( Fig. 2c,d ). These spectral shifts are consistent with the trend observed for gold/silver nanodisks that result from an increase in the dipole moment [8] , [29] . Electric field enhancement plots at the spectral dips for the selected pixels are shown in Fig. 2e,f , respectively, for y - and x -polarized illuminations. Here, the pixel resonances were observed at the dips in the reflection spectra corresponding to light absorption in the metal ellipses, corroborated by Poynting vectors directed into the nanostructures [8] . For an elliptical pixel with L y =190 nm and L x =100 nm, strong field enhancements occurred at the periphery of the ellipses for both orthogonally polarized illuminations ( Fig. 2e,f ). In contrast to light polarized along the axis in which the dimension of the ellipse was varied, we expected that the colour of scattered light polarized along the dimension that is held constant to remain unchanged. Indeed, we observed that different pixel arrays exhibited similar colours when light is polarized along the dimension that was held constant, that is, horizontal rows under y -polarized illumination ( Fig. 2a ) and vertical columns under x -polarized illumination ( Fig. 2b ). For example, within each row ( L y =190 nm), a constant colour with a resonance at ~713 nm was observed as L x was increased from 100 to 190 nm under y -polarized illumination ( Fig. 2a ). In our previous work, it was shown that similar colours could be generated for pixels with the same fill factor (defined here as L y /pitch for the y axis of the ellipses) [8] . Similarly, we show here that by maintaining L y and the fill factor along the y axis, their observed resonances remain almost constant despite variations in the orthogonal axis. Therefore, the colours are determined almost purely by the dimension of the ellipse axis parallel to the polarization direction, that is, the L y axis for y -polarized light illumination. However, despite fixing the dimensions of the ellipses along the polarization of the light, cross-talk resulted in slight tonal changes. Cross-talk manifested as minute shifts (<10 nm) in the spectra for horizontal rows in the colour palette illuminated under y -polarized light ( Fig. 2c ), which occurred owing to changes in the oscillator strength as dimensions are varied in the orthogonal axis. The effect of cross-talk can be reduced using coupled nanosquare dimers that are designed to operate differently from the ellipses. Here, we varied the gap size and nanosquare width. When the incident illumination is polarized along the axis of two closely spaced nanosquares, a coupled-dipole mode is excited with strong fields within the gap [30] . In the orthogonal direction, another resonance at a different wavelength is excited with the field localized at the aligned edges of the nanosquares, producing a slightly different colour. As this mode is not affected by plasmon coupling [31] , their corresponding spectra are independent of gap size. Therefore, these coupled nanosquares will experience less cross-talk compared with the ellipses. The disadvantage of dimer structures, however, lies in the relatively narrower span of colours that can be achieved owing to coupling, that is, by varying the gap size. To investigate the full palette of colours that can be achieved, the widths, w of the dimers were varied from 75 to 120 nm in 5 nm increments, with gaps varied from 25 to 80 nm in 5 nm increments. With the polarization along the dipole axis, a redshift in the spectrum is seen with a reduction in gap size due to plasmon coupling ( Fig. 3d ). In addition, as a result of this coupling, a gap width of ~50 nm or smaller is required before a notable colour change can be observed. The redshift in the dip of the reflection spectra occurs ( Fig. 3b ) for decreasing gap sizes is because of the increase in the capacitance within gaps as the nanosquares are brought closer together [31] , [32] . These colour differences are accompanied by changes in the electric field strength ( Fig. 3d,f ) with stronger coupling in smaller gaps (that is, towards g =25 nm; ref. 31 ) Conversely, as gaps are increased beyond 60 nm, coupling becomes negligible and the nanosquare pairs start to resemble single, isolated square structures that are polarization independent ( Fig. 3d,f and Supplementary Fig. 2c,d ). 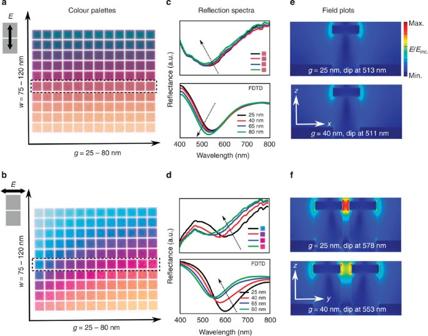Figure 3: Optical micrographs and spectral analyses for coupled nanosquare pixels with varying dimensionswand gapsg. (a,b) Optical images of colour palettes illuminated undery- andxpolarized light. Each 8 × 8 μm pixel array was spaced 1 μm away from the neighbouring pixel and comprised a square lattice of 20 × 20 nanoposts with periodd=400 nm. (c,d) Measured and simulated reflection spectra under orthogonal illumination where arrows indicate decreasing gap sizesg. (e,f) Electric field enhancement plots (w=95 nm,g=25, 40 nm). Panelsa,c,eandb,d,fcorrespond to results obtained undery- andxpolarization, respectively. Figure 3: Optical micrographs and spectral analyses for coupled nanosquare pixels with varying dimensions w and gaps g . ( a , b ) Optical images of colour palettes illuminated under y - and x polarized light. Each 8 × 8 μm pixel array was spaced 1 μm away from the neighbouring pixel and comprised a square lattice of 20 × 20 nanoposts with period d =400 nm. ( c , d ) Measured and simulated reflection spectra under orthogonal illumination where arrows indicate decreasing gap sizes g . ( e , f ) Electric field enhancement plots ( w =95 nm, g =25, 40 nm). Panels a , c , e and b , d , f correspond to results obtained under y - and x polarization, respectively. Full size image In the case where light is polarized perpendicular to the dipole axis, colours remain insensitive to gap widths as the gap capacitances of the coupled nanosquares are not charged in the associated resonant mode. This gap size independence is confirmed in the spectral analyses ( Fig. 3c ) corresponding to the row of the colour palette ( w =95 nm) highlighted by dotted lines ( Fig. 3a ). Coupled nanosquares of these widths, for example, produce a brown colour with a spectral dip at ~524 nm under y -polarized illumination, with no change in the electric field surrounding the pixels ( Fig. 3c ). In the orthogonal polarization, a range of blues and purples, with dips at ~603 nm ( g =25 nm) and ~531 nm ( g =80 nm) were observed instead ( Fig. 3d,e ). For both types of pixels investigated, experimental spectra demonstrated good qualitative agreement with finite difference time domain (FDTD) simulations where a redshift in the spectral dips was be observed with increasing dimensions (that is, L x and L y ) for the ellipses ( Fig. 2c,d ), consistent with the trends observed for gold/silver nanodisks [8] , [29] , and with decreasing gap widths g for the nanosquares ( Fig. 3c,d ) [31] . As the size of the nanostructure increases, retardation effects cause a redshift in the resonance. The increase in the extinction cross-section or oscillator strength then gives rise to the larger dip in the spectra owing to the larger dipole moment induced by the increased dimension [8] , [29] . We note that additional reflection dips at 450 and 400 nm are observed only from the measured spectrum in Figs 2c and 3d , indicating that the nature of the resonances observed here is more complex, involving the consideration of resonances that were not captured in simulations. For example, given the pixel periodicity of 400 nm, scattering into surface lattice resonances from free space wavelengths at comparable but slightly longer wavelengths could occur. In the experiments, the illumination was not entirely normal to the sample and incorporated tilt angles that could excite additional resonances that give rise to the dips in the measured spectra. These effects were not observed in the simulations, in which only normal incidence was considered. A careful and detailed study of this effect would be worthwhile but is beyond the scope of the current manuscript. Furthermore, the trends observed for the experimental spectra nevertheless showed good agreement with computational simulations. Cross-talk quantification and colour resolution tests Low cross-talk and good colour separation are crucial for minimizing the mixing of images intended for two orthogonal polarizations despite their overlay on a common printed area. To quantify the cross-talk observed, red–green–blue (RGB) values of these pixels were compared with that of a disk or nanosquare spaced far apart (that is, isolated nanostructures). RGB differences are defined as ( R − R c ) 2 +( G − G c ) 2 +( B − B c ) 2 , where R , G and B refers to values for the elliptical or nanosquare pixels, and R c , G c and B c , refer to values for either a reference disk of a diameter equal to the unchanged axis of the ellipse or nanosquares of the same widths with a gap of 80 nm. Colour palettes in Figs 2 and 3 reveal superior colour generation in the ellipses with 10 different polarization-dependent colours compared with ~2–3 colours using the nanosquares. However, ellipses exhibit more observable cross-talk compared with the coupled nanosquares as shown in Fig. 4a . For example, ellipses with L y =150 nm had RGB differences >50 (for L x =100–190 nm), while nanosquares with w =120 nm had an average RGB difference of ~30. Given their gap-dependent colour tuning for light polarized along the dipole axis, and gap-independent mode for the orthogonal polarization, nanosquare experience a lower cross-talk (at the cost of a narrower range of colours). These attributes can be useful in printing two distinct images in different colours onto the same area that can be decoupled with high image clarity under orthogonal polarizations. To highlight the advantages of each pixel type, we will demonstrate in a later section, the use of both pixels for printing dual-image embedded microprints and a stereoscopic image. It should be noted that while this work focuses on colour pixels with the pitch fixed at 400 nm, different colour tones can be generated through variation of the pitch [27] . Although the colour tones generated typically appear more ‘intense’ for pixels with smaller pitch, surface plasmon coupling owing to the close proximity of nanostructures might result in increased cross-talk. 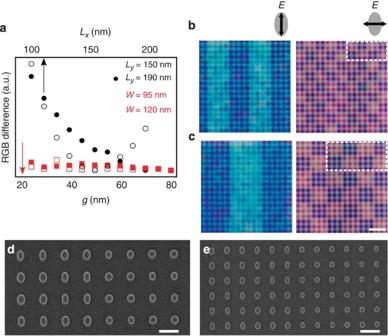Figure 4: RGB difference cross-talk variable plots and full-colour pixel resolution test pattern images. (a) RGB values for elliptical and coupled nanosquare pixels normalized to that of a disk of which the diameter is of the same size asLyof the ellipse, or nanosquares of widthswwith gapsg=80 nm. (b,c) Colour pixel resolution test structures consisting of patterns in alternating colours (b) at and (c) approaching the optical diffraction limit illuminated undery- andx-polarized light. Scale bars, 2 μm. (d,e) SEM images of the regions indicated by the dotted boxes inb,c, respectively. Scale bars, 500 nm. Note the slight differences in dimensions that resulted in the colour variants in thex- andypolarizations. Figure 4: RGB difference cross-talk variable plots and full-colour pixel resolution test pattern images. ( a ) RGB values for elliptical and coupled nanosquare pixels normalized to that of a disk of which the diameter is of the same size as L y of the ellipse, or nanosquares of widths w with gaps g =80 nm. ( b , c ) Colour pixel resolution test structures consisting of patterns in alternating colours ( b ) at and ( c ) approaching the optical diffraction limit illuminated under y - and x -polarized light. Scale bars, 2 μm. ( d , e ) SEM images of the regions indicated by the dotted boxes in b , c , respectively. Scale bars, 500 nm. Note the slight differences in dimensions that resulted in the colour variants in the x - and y polarizations. Full size image To investigate the resolution of these colour pixels, a set of resolution test structures was fabricated using elliptical pixels. Each pattern consists of a 2 × 2 ( Fig. 4b ) or 3 × 3 ( Fig. 4c ) array of ellipses where a single ellipse forms a pixel of colour on a 400-nm-pitch grid. Under y -polarized light illumination, the patterns exhibit colour stripes. Under x -polarized light illumination, a distinctly different set of alternating colours in a checkerboard pattern is observed instead. We note that in Fig. 4c , both the grid of individual ellipses and the checkerboard pattern are clearly visible. Therefore, each individual ellipse stands alone as a single colour element giving rise to print resolutions at the single-nanostructure level, where even minor changes in pixel geometry due to fabrication imperfections are observable as minor colour variations. Such polarization-dependent microprints open up the possibility of achieving two different diffraction patterns (that is, a grating and a checkerboard) depending on the polarization of incident illumination and could find application in areas such as holography. Dual-image embedded microprints and stereoscopic image The polarization-dependent spectral tunability of these biaxial colour pixels allow for the encoding of two sets of colour information within a single layer on a substrate. We demonstrate the printing of two overlaid images using elliptical and coupled nanosquare pixels with the colours palettes derived in Figs 2a,b and 3a,b . As shown in Fig. 5a,b , the microprints were designed to reveal different images when illuminated under orthogonal polarizations: Under y polarization, a square is observed while a cross is revealed under x polarization. Notably, this approach can be extended to encode multiple images (that is, more than two images). For example, circularly asymmetric nanostructures could be used so that in addition to the x – y polarization control demonstrated here, one can extract further information in the circularly polarized dimension. The microprint formed from nanosquares ( Fig. 5b ) shows better cross-talk suppression compared with the prints with ellipses where a faint outline of a square can still be discerned in the image of the cross ( Fig. 5a ). Note that these pixels exhibit tolerance to fabrication errors introduced during the lithographic step: pixels comprising ellipses formed with rough edges maintained polarization-sensitivity such that each image was still revealed only under the design polarization illumination as shown in Supplementary Fig. 3 . 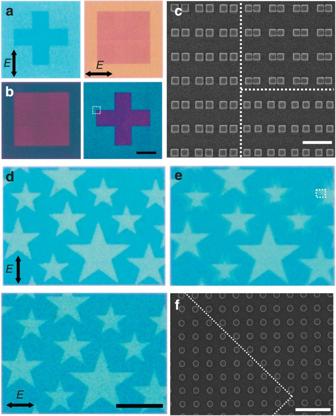Figure 5: Dual-image embedded plasmonic colour microprints and a stereoscopic image. Optical microprints of a square and a cross printed onto the same area formed from (a) ellipses and (b) coupled nanosquare pixels illuminated underx- andy-polarized light. Scale bar, 20 μm. (c) SEM image of the region indicated by the dotted box inb. Regions comprising nanosquares of the same dimensions and gap widths are separated by the dotted lines. (d) Overlaid images decoupled by polarizers. Scale bar, 20 μm. (e) Overlay of images indforms a stereoscopic image with depth perception. (f) SEM image of the region indicated by the dotted box ine. Each pixel in these microprints was a 400 × 400 nm square. Scale bar, 1 μm. Figure 5: Dual-image embedded plasmonic colour microprints and a stereoscopic image. Optical microprints of a square and a cross printed onto the same area formed from ( a ) ellipses and ( b ) coupled nanosquare pixels illuminated under x - and y -polarized light. Scale bar, 20 μm. ( c ) SEM image of the region indicated by the dotted box in b . Regions comprising nanosquares of the same dimensions and gap widths are separated by the dotted lines. ( d ) Overlaid images decoupled by polarizers. Scale bar, 20 μm. ( e ) Overlay of images in d forms a stereoscopic image with depth perception. ( f ) SEM image of the region indicated by the dotted box in e . Each pixel in these microprints was a 400 × 400 nm square. Scale bar, 1 μm. Full size image To highlight the potential of using these polarization-sensitive pixels in high-resolution 3D full-colour elements, we demonstrate a stereoscopic plasmonic colour print composed of images of objects viewed from laterally offset positions formed on the same area. Here, elliptical pixels were specifically chosen to create the stereoscopic print given their broad range of colours and tones. The microprint pattern of stars decoupled by polarizers is shown in Fig. 5d . By viewing the overlaid microprint through polarizers with orthogonal orientation on the eye pieces, a unique image is presented to each eye. The separate images are overlaid in Fig. 5e to provide a 3D representation of the image when viewed optically. In particular, the smaller stars are displaced by larger distances to give the impression of them being further away from the viewer than the larger stars. Judicious choice of the pixel elements, that is, choosing similar colours for the stars and the background enabled total cross-talk suppression in this image. Figure 5f shows the scanning electron microscope (SEM) image of the region indicated by the dotted box in Fig. 5e , where regions comprising ellipses of the same dimensions are indicated by the dotted lines. With this, we have printed the first stereoscopic plasmonic colour image composed of offset images that can only be decoupled through the use of polarizers. In comparison with conventional stereoimages, these 3D plasmonic analogues provide superior resolution in full-colour, and could find applications in robust anti-forgery elements as well as novel 3D colour imaging and displays. We have presented a single-layer architecture of polarization-dependent reflective colour pixels, able to be independently tuned with resolutions approaching the optical diffraction limit. Two types of biaxial aluminium nanostructures—ellipses and coupled nanosquare dimers—were investigated. The ellipses had a noticeably broader range of polarization-dependent colours but higher cross-talk than the coupled nanosquares. Studies into the pixels tilted at different angles as shown in Supplementary Fig. 4 revealed colour invariance for tilt angles smaller than 20°, and gradual colour changes for tilt angles larger than 25°. Given the large pitch (400 nm) of the pixels used here, the colour change beyond tilt angles larger than 25° is not unexpected. Colours from pixels with smaller periodicities, that is, smaller than 400 nm, are anticipated to be angle insensitive, consistent with studies performed on similar nanohole and disk structures [33] . Our approach enables the printing of two overlaid full-colour images that can be independently decoded when viewed through a polarizing filter—a powerful capability that could potentially be extended to encoding multiple images (that is, through the use of circularly asymmetric nanostructures) or generating stereoscopic microprints. Importantly, the choice of aluminium as the functional material in the pixel design alleviates costs associated with other noble metals (that is, gold) and improves pixel shelf-life and durability compared with those fabricated from silver. In addition, the polarization-sensitive colour pixels reported in this manuscript produce distinct SPP-induced changes in spectra under orthogonal polarizations of incident light. Therefore, it can provide a viable recording material as each nanostructure now holds two sets of information, one for each polarization. This feature of the pixels enables the encoding of information in different colours and polarization [17] , now with a single layer and lithographic step. As such, with the ease of generating a full-colour high-resolution image that can markedly change its appearance under orthogonal polarization illuminations, such polarization-dependent encoding could pave the way for new, effective colour display elements, and have significant impact for realizing advanced security elements or high-density spectrally encoded optical data storage applications. Electron beam lithography Colour information in the microprints was encoded in the form of nanostructure dimension and position by use of MATLAB (The Mathworks Inc.) for fabrication in EBL. To achieve this, negative-tone electron beam resist HSQ (XR-1541-006, Dow Corning, 6% concentration in MIBK solvent) was spin-coated at 4,000 r.p.m. onto silicon substrates to a thickness of ~95 nm. Baking of the resist was not performed so as to avoid thermally induced crosslinking that reduces resolution of the resist. Computer-generated pattern layouts defining arrays of ellipses or closely spaced nanosquares with diameters or widths ranging from 90 to 190 nm in 10 nm increments and 75–120 nm in 5 nm increments, respectively, spaced 400 nm apart were input into the lithography system for writing. EBL was performed using an Elionix ELS-7000 EBL system (Elionix Inc.) with an accelerating voltage of 100 kV and a beam current of 500 pA. A write field of 150 × 150 μm with an exposure step size of 2.5 nm was used. A dose of 12 mC cm −2 was used for all exposures. No proximity-effect corrections were performed for the exposures. To form well-defined nanostructures with near-vertical sidewalls, a high-contrast development process was used [34] . Unexposed regions of HSQ were removed by immersing the samples in an aqueous formulation of 1% NaOH, 4% NaCl in deionized water for 60 s, followed by rinsing under running deionized water for 30 s. Finally, the samples were blow-dried using N 2 . Metal deposition Metal deposition was performed using an electron beam evaporator (Explorer Coating System, Denton Vacuum Inc.) at a working pressure of ~1 × 10 −6 Torr. A 20-nm-thick layer of aluminium was deposited onto the samples at the rate of 1.5 Å s −1 . During the evaporation process, the sample chamber was kept at a constant temperature of 20 °C and the sample holder was rotated at 50 r.p.m. to maintain uniform deposition. The fabricated structures were characterized and imaged using an Elionix ESM-9000 (Elionix Inc.) scanning electron microscope with an accelerating voltage of 10 kV and a working distance of 5 mm. Optical measurements Bright-field optical images and reflection spectra measurements of the colour palettes were obtained to investigate the optical responses of the fabricated structures. Extinction spectrometry in reflection mode was performed using a UV-visible-near infrared (NIR) microspectrophotometer (CRAIC Technology Inc.) at normal incidence with a 75-W broadband xenon source. White light passed through an objective lens (36 × 0.5 numerical aperture) and polarized parallel and perpendicular to the colour pixels illuminated the samples at normal incidence to the substrate. Using a variable aperture set to a detecting area of 3.5 × 3.5 μm, reflected light ( λ =400–800 nm) was collected through the same objective and back into the spectrometer and CCD camera. Reflection measurements were normalized with respect to an aluminium mirror. Optical images were captured using a conventional upright bright-field reflection microscope (Olympus MX61, Olympus Inc.) equipped with a digital camera (SC30 Olympus). Images of samples were magnified by an objective lens (Olympus Mplan 50 × 0.8 numerical aperture (NA)) and polarized in both orthogonal directions in order to observe the different colours exhibited under different polarization states. Post-processing steps (background normalization) for the optical images were performed using ImageJ (National Institutes of Health (NIH), MD, USA). Numerical simulations The optical responses of the colour pixels were modelled using FDTD (Lumerical FDTD Solutions, version 8.6.2; ref. 35 ) Individual pixels with different dimensions and width of gaps formed between adjacent nanostructures (in the case of the coupled nanosquare pixels) were simulated. A constant refractive index of 1.4 was used for HSQ. The complex refractive indices of aluminium and silicon were taken from Palik [36] . Each pixel was illuminated with a normal incident plane wave using a total field scattered field source in the spectral range λ =400–800 nm in increment step sizes of 1 nm. Perfectly matched layer boundary conditions were defined at a minimal of half a wavelength away for each single pixel. To calculate the reflection spectra, the absorption and transmission were subtracted from the total incident power simulated. How to cite this article: Goh, X. M. et al . Three-dimensional plasmonic stereoscopic prints in full colour. Nat. Commun. 5:5361 doi: 10.1038/ncomms6361 (2014).